A toolbox of oligopeptide-modified polymers for tailored elastomers Biomaterials are constructed from limited sets of building blocks but exhibit extraordinary and versatile properties, because hierarchical structure formation lets them employ identical supramolecular motifs for different purposes. Here we exert a similar degree of structural control in synthetic supramolecular elastomers and thus tailor them for a broad range of thermomechanical properties. We show that oligopeptide-terminated polymers selectively self-assemble into small aggregates or nanofibrils, depending on the length of the oligopeptides. This process is self-sorting if differently long oligopeptides are combined so that different nanostructures coexist in bulk mixtures. Blends of polymers with oligopeptides matching in length furnish reinforced elastomers that exhibit shear moduli one order of magnitude higher than the parent polymers. By contrast, novel interpenetrating supramolecular networks that display excellent vibration damping properties are obtained from blends comprising non-matching oligopeptides or unmodified polymers. Hence, blends of oligopeptide-modified polymers constitute a toolbox for tailored elastomers with versatile properties. Structural proteins are constructed from a finite number of amino acids and their self-organization relies on a limited set of supramolecular interactions. Nevertheless, they constitute the basis for a broad array of different structure materials with tailored mechanical properties [1] , [2] . This versatility is achieved by structure formation on several levels of the structural hierarchy [3] , [4] . The different strength, toughness and extensibility of various types of silk materials, for instance, result from a combination of highly ordered β-sheet nanofibrils from alanine-rich segments as a reinforcement [5] , [6] , a ‘string of beads’ of short single β-sheet tapes for energy dissipation on mechanical load [5] , [7] , [8] , [9] and amorphous domains that provide elasticity [6] , [10] . The silk proteins’ sophisticated structure and carefully guided folding, self-organization and phase segregation during the spinning process allows these different structural motifs to coexist in the final material. In this way, the versatile properties of different types of silk materials are precisely tailored according to their function [11] , [12] , [13] . Inspired by this example of nature’s design principles, the selective formation of one-dimensional nanostructures from β-sheet-forming oligopeptides and oligopeptide-modified polymers has been extensively investigated [14] , [15] , [16] , [17] , [18] , [19] , [20] , [21] , [22] , [23] , [24] , [25] , [26] , [27] , [28] . However, the thermomechanical properties of the corresponding bulk materials have rarely been studied in much detail [29] , [30] , [31] . Supramolecular materials from polymers with other types of hydrogen-bonded end groups have frequently been used to obtain thermoplastic elastomers with superior processing behaviour at elevated temperatures [32] , [33] , [34] , [35] , [36] , [37] , [38] , [39] . In these materials, network formation by non-covalent interactions allows for dynamic reorganization processes, which is relevant for self-healing or thermoresponsive materials [40] , [41] . Here we provide the first example of exploiting the hierarchical structure formation of oligopeptides to systematically tailor the thermomechanical properties of polymer materials. To this end, we investigate a series of novel supramolecular materials from mixtures of oligopeptide-modified and unmodified poly(isobutylene)s (PIBs). Extending on previous examples of supramolecular networks [32] , [33] , [34] , [35] , [36] , [37] , [38] , [39] , these materials show an additional formation of defined nanostructures. The length-dependent aggregation of the oligopeptides results in the formation of either small hydrogen-bonded aggregates that serve as physical cross-links in the material, or mixtures of single β-sheet tapes and stacked β-sheet nanofibrils that provide a secondary network and serve as a reinforcement ( Fig. 1 ). This self-assembly is ‘self-sorting’ in the sense that nanostructures obtained from differently long oligopeptide end groups coexist in the bulk materials. Thus, the molecular level control over this process allows us to use mixtures of molecules to design materials with vastly different property profiles, even if their components have similar molecular structures or thermomechanical properties. As a result, mixtures of molecules with identical oligopeptide segments give rise to elastomers that are inherently reinforced with the β-sheet tapes or nanofibrils and exhibit significantly higher moduli than the parent polymers, as well as excellent processing properties at elevated temperatures. By contrast, blends of derivatives with non-matching oligopeptides or unmodified polymers form novel ‘interpenetrating supramolecular networks’. Some of the latter materials may be of interest as ‘self-healing’ elastomers while others showed promising performance in mechanical-vibration damping, which is relevant for automotive and aerospace applications [42] . In this way, blends of polymers modified with short β-sheet forming oligopeptide termini constitute a simple yet highly versatile toolbox that gives rise to soft elastomers with tailored thermomechanical properties. 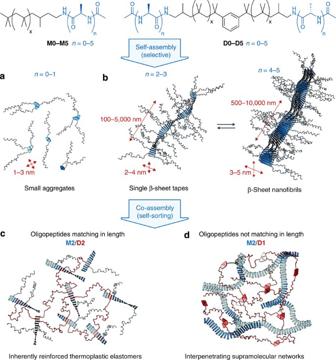Figure 1: Schematic illustration of the selective self-assembly and self-sorting co-assembly processes. Depending on the oligopeptide length, the monofunctional oligo(L-alanine)-modified PIBsM0–M5(n=0–5;x≈20) as well as the corresponding difunctional derivativesD0–D5(n=0–5;x≈20) self-organize into (a) small hydrogen-bonded aggregates or (b) stacked β-sheet fibrils, accompanied by single β-sheet tapes. The coexistence of these nanostructures in blends of molecules with different oligopeptide termini results in (c) ‘inherently reinforced thermoplastic elastomers’ or (d) ‘interpenetrating supramolecular networks’. Figure 1: Schematic illustration of the selective self-assembly and self-sorting co-assembly processes. Depending on the oligopeptide length, the monofunctional oligo( L -alanine)-modified PIBs M0–M5 ( n =0–5; x ≈20) as well as the corresponding difunctional derivatives D0–D5 ( n =0–5; x ≈20) self-organize into ( a ) small hydrogen-bonded aggregates or ( b ) stacked β-sheet fibrils, accompanied by single β-sheet tapes. The coexistence of these nanostructures in blends of molecules with different oligopeptide termini results in ( c ) ‘inherently reinforced thermoplastic elastomers’ or ( d ) ‘interpenetrating supramolecular networks’. Full size image Selective self-assembly in solution and in bulk The monofunctional oligo( L -alanine)-terminated polymers M0–M5 and their difunctional siblings D0–D5 ( Fig. 1 ) were synthesized by simple peptide-coupling procedures ( Supplementary Fig. 1 ). Repeated precipitation procedures furnished the polydisperse compounds in chemically pure form with complete end-group functionalization. The obtained oligopeptide-modified polymers exhibited distinctly different aggregation properties, depending on the length of the oligo( L -alanine) segment ( n =0–5 alanine residues). An analysis of peak positions and intensities in the solution-phase or solid-state infrared spectroscopy ( Fig. 2a–c and Supplementary Figs 2–4 ) proved that the end groups in M0–M1 and D0–D1 were too short to induce β-sheet formation either in the bulk or in solution; M2–M3 and D2–D3 formed antiparallel β-sheets predominantly in the bulk materials; and M4–M5 and D4–D5 gave rise to highly ordered and strongly aggregated β-sheets structures both in bulk and in solution. Atomic force microscopy (AFM) imaging ( Fig. 2d and Supplementary Fig. 5 ) then established an excellent link to the corresponding nanoscopic morphologies for the monofunctional derivatives M0–M5 . Thus, rigid and many micrometre-long fibrils with diameters of a few nanometres were observed for M5 and M4 , independent of whether highly oriented pyrolytic graphite (HOPG) or more polar SiO 2 substrates were used. These nanofibrils were formed from stacked β-sheets and the heights of nanofibrils from M4 and M5 in the AFM images suggested that they comprised two to four and four to six stacked β-sheet tapes, respectively. Moreover, they remained distinguishable entities even inside larger ‘bundles’ visible in the AFM images ( Supplementary Figs 5 and 6 ). Moreover, a second population of thinner aggregates was observed on HOPG that, based on their dimensions, were assigned to single β-sheet tapes. M3 gave rise to long tape-like features on HOPG, and for M2 we observed laterally aggregated tape-like features on HOPG with lengths on the order of a few hundred nanometres. Consistent with infrared spectroscopy, the epitaxial orientation of these tape-like features on HOPG and their absence on the more polar SiO 2 substrates suggested that they had not been present in solution but were formed in the course of solvent evaporation. 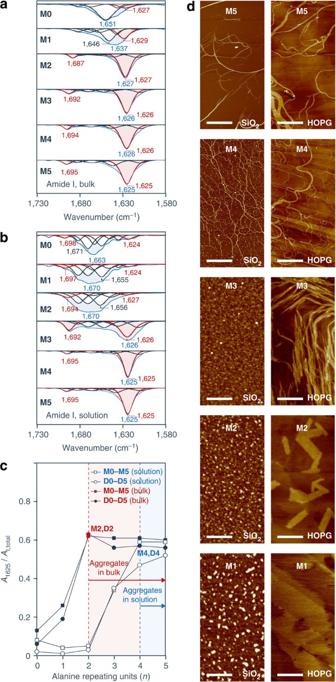Figure 2: Nanostructure formation in solution and in bulk. Amide I regions of (a) the solid-state and (b) the solution-phase infrared spectra ofM0–M5, and the constituent absorption bands obtained by peak deconvolution. Bulk infrared spectra ofM2–M5as well as solution-phase spectra ofM4–M5exhibited a sharp amide I absorption at 1,625–1,627 cm–1(half-height width 14–17 cm−1) accompanied with a secondary absorption at 1,687–1,695 cm−1, consistent with the presence of antiparallel β-sheet structures. (c) Plots of the relative peak areaA1,625/AI,totalof the absorption bands at around 1,625–1,630 cm−1showed thatM2–M5andD2–D5in bulk, as well asM4–M5andD4–D5in solution were strongly aggregated. (d) AFM images ofM1–M5spin-coated from tetrachloroethane solution onto SiO2(left) or HOPG (right) substrates revealed the formation of fibrils forM5on both substrates (scale bars, 300 nm forM1–M3and 2 μm forM4–M5). The fibrils exhibited a width of 7.0 (±0.1) nm and a uniform height of 3.5 (±0.8) nm, suggesting they were formed from four to six stacked β-sheet tapes. Fibrils ofM4on both substrates were less defined and 2.1 (±0.9) nm in height, consistent with two to four stacked β-sheet tapes. A second population of thin aggregates (8–10 nm in width, 0.4–0.6 nm in height) was observed on HOPG (but not SiO2) that were assigned to single β-sheet tapes.M3gave rise to long flexible fibrils or tapes (0.7–1.2 nm in height, consistent with one to two β-sheet tapes) only on HOPG. In the case ofM2, laterally aggregated, short tape-like features (height 0.7 nm) with lengths of several hundred nanometres were observed on HOPG. No defined aggregates but continuous films or drop-like features were observed forM1. SeeSupplementary Figs 2–6for details on infrared spectra, peak deconvolution and AFM imaging ofM0–M5andD0–D5. Figure 2: Nanostructure formation in solution and in bulk. Amide I regions of ( a ) the solid-state and ( b ) the solution-phase infrared spectra of M0–M5 , and the constituent absorption bands obtained by peak deconvolution. Bulk infrared spectra of M2–M5 as well as solution-phase spectra of M4–M5 exhibited a sharp amide I absorption at 1,625–1,627 cm –1 (half-height width 14–17 cm −1 ) accompanied with a secondary absorption at 1,687–1,695 cm −1 , consistent with the presence of antiparallel β-sheet structures. ( c ) Plots of the relative peak area A 1,625 / A I,total of the absorption bands at around 1,625–1,630 cm −1 showed that M2–M5 and D2–D5 in bulk, as well as M4–M5 and D4–D5 in solution were strongly aggregated. ( d ) AFM images of M1–M5 spin-coated from tetrachloroethane solution onto SiO 2 (left) or HOPG (right) substrates revealed the formation of fibrils for M5 on both substrates (scale bars, 300 nm for M1–M3 and 2 μm for M4–M5 ). The fibrils exhibited a width of 7.0 (±0.1) nm and a uniform height of 3.5 (±0.8) nm, suggesting they were formed from four to six stacked β-sheet tapes. Fibrils of M4 on both substrates were less defined and 2.1 (±0.9) nm in height, consistent with two to four stacked β-sheet tapes. A second population of thin aggregates (8–10 nm in width, 0.4–0.6 nm in height) was observed on HOPG (but not SiO 2 ) that were assigned to single β-sheet tapes. M3 gave rise to long flexible fibrils or tapes (0.7–1.2 nm in height, consistent with one to two β-sheet tapes) only on HOPG. In the case of M2 , laterally aggregated, short tape-like features (height 0.7 nm) with lengths of several hundred nanometres were observed on HOPG. No defined aggregates but continuous films or drop-like features were observed for M1 . See Supplementary Figs 2–6 for details on infrared spectra, peak deconvolution and AFM imaging of M0–M5 and D0–D5 . Full size image X-ray diffraction (XRD) and small-angle X-ray scattering (SAXS) confirmed that this length-dependent formation of different types of nanostructures was also present in the bulk materials ( Fig. 3a–c ). The XRD patterns of all derivatives M0 – M5 showed a main reflection at a spacing of 6.0–6.4 Å that can be attributed to the short-range order of the PIB segments in their preferred 8 3 helical conformation [43] , [44] . A second reflection at a spacing of 4.2–4.4 Å was observed only for M2 – M5 . This peak can be assigned to the intermolecular spacing between oligopeptides within a β-sheet tape. Notably, however, it is significantly smaller than the typical value of ~4.8 Å observed in proteins, due to strong hydrogen bonding in the hydrophobic matrix [20] , [30] , [45] , [46] . Moreover, M2 – M5 exhibited an additional reflection at a spacing of 5.3–5.4 Å, corresponding to the intersheet distance between stacked β-sheets observed in poly( L -alanine) [45] , spider silk (5.30 Å) [47] or related materials [20] , [30] , [46] ( Fig. 3a ). From the full-width at half-maximum of the latter reflection at 5.3–5.4 Å in the case of M2–M5 , one can determine a crystallite size on the order of 24–27 Å using the Scherrer equation, which roughly indicates that the superstructures formed by these derivatives in the bulk comprised approximately four to five stacked β-sheet tapes. Interestingly, the intensity of this reflection normalized with the intensity of the PIB reflection increased in two steps from M0–M1 to M2–M3 and finally M4–M5 , suggesting that the relative concentration of stacked β-sheet structures was distinctly different for these three groups of compounds ( Fig. 3b ). 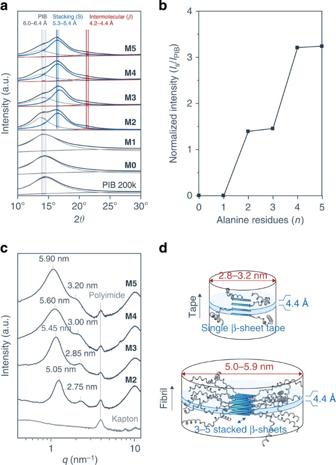Figure 3: Hierarchical structure formation according to XRD. (a) X-ray diffractograms ofM0–M5along with the deconvolution of the three main reflections at 2θ=13.7°–14.7° (short-range order of PIB), 16.1°–16.8° (β-sheet stacking) and around 21° (intermolecular distance within β-sheets). (b) The normalized intensity of the reflection at 2θ=16.1°–16.8° (relative to the one at 13.7°–14.7°) as a function of the number ofL-alanine repeating unitsn. (c) SAXS curves of samples ofM0–M5on a polyimide support (scattering peak atq=3.95 nm−1due to the support). (d) Schematic illustrations of cross-sections of single β-sheet tapes or nanofibrils composed of three to five stacked β-sheet tapes, and the volumes of cylinder slices (blue) with a thickness corresponding to the intermolecular distance. Figure 3: Hierarchical structure formation according to XRD. ( a ) X-ray diffractograms of M0–M5 along with the deconvolution of the three main reflections at 2 θ =13.7°–14.7° (short-range order of PIB), 16.1°–16.8° (β-sheet stacking) and around 21° (intermolecular distance within β-sheets). ( b ) The normalized intensity of the reflection at 2 θ =16.1°–16.8° (relative to the one at 13.7°–14.7°) as a function of the number of L -alanine repeating units n . ( c ) SAXS curves of samples of M0–M5 on a polyimide support (scattering peak at q =3.95 nm −1 due to the support). ( d ) Schematic illustrations of cross-sections of single β-sheet tapes or nanofibrils composed of three to five stacked β-sheet tapes, and the volumes of cylinder slices (blue) with a thickness corresponding to the intermolecular distance. Full size image In the SAXS region ( Fig. 3c ), the compounds exhibited two peaks at 5.05–5.90 and 2.75–3.20 nm that successively increased in spacing from M2–M5 . From these two d spacings, one can calculate the volumes of the respective slices of the cylindrical envelopes with a thickness corresponding to the intermolecular distance (4.2–4.4 Å) to be in the range of 8,410–11,480 Å 3 and 1,740–1,970 Å 3 for M2–M5 ( Fig. 3d and Supplementary Table 1 ). Comparing these values with the molecular Van der Waals volumes of 2,510–3,380 Å 3 for M2–M5 allowed us to conclude that the SAXS peaks at 2.75–3.20 nm originated from single β-sheet tape structures, while those at 5.05–5.90 nm corresponded to nanofibrils comprising three to five stacked β-sheet tapes ( Fig. 3d ), qualitatively also taking into account excluded volume and consistent with the AFM and XRD data. As will be shown in the following sections, this coexistence of different nanostructures in binary mixtures of M0–M5 and D0–D5 , as well as their blends with non-functionalized PIB is the key for tailoring supramolecular materials with various property profiles. Thermomechanical properties of oligopeptide-modified polymers Shear rheology on the monofunctional derivatives M0–M5 in comparison with unmodified PIB revealed a drastic transition of mechanical properties from a moderately viscous liquid ( M0–M1 ) to a rubbery behaviour ( M4–M5 ) as a function of the number of n alanine residues ( Fig. 4a,b and Supplementary Figs 7–10 ). Starting with the β-sheet tape-forming derivative M2 , the materials already exhibited shear moduli exceeding those of high-molecular weight (MW) PIB, which is remarkable considering that the MW of the attached polymer (1,200 g mol −1 ) was far below the entanglement length of PIB (≈15,000 g mol −1 ) and the monofunctional (as opposed to the difunctional) derivatives could not form hydrogen-bonded networks. The materials became rubbery in the case of M4 and M5 , because the stable β-sheet-like tapes and nanofibrils themselves gave rise to an entangled network. Moreover, the storage and loss moduli at 1 rad s −1 within the series leveled off towards G′ ≈0.6 MPa and G″ ≈0.06 MPa for M5 ( Supplementary Fig. 10 ), indicating that a further increase of the oligopeptide length would not substantially affect the materials’ mechanical properties anymore. The network-forming difunctional derivatives D0–D2 showed even more drastic changes in mechanical properties as a function of oligopeptide length. D1 , for instance, exhibited a rheological behaviour and moduli very similar to PIB with moderate MW (75,000 g mol −1 ), with an entanglement point in a similar frequency range at room temperature. D2 was already a brittle hard solid ( G′ =2 MPa) and the higher homologues could not even be investigated by shear rheology anymore. Although the general notion of a mechanical reinforcement is certainly well in line with previous reports on supramolecular networks [32] , [35] , including modified PIBs [36] , [37] , [38] , [39] , the observed drastic dependence of aggregation behaviour and mechanical properties on the number of hydrogen-bonding sites allowed for further tailoring of the materials’ thermomechanical properties. To this end, binary blends of monofunctional and difunctional derivatives with ‘matching’ oligopeptide segments were found to give rise to supramolecular networks that were ‘inherently reinforced’ by the incorporated β-sheet aggregates. Thermogravimetric analysis, differential scanning calorimetry (DSC) and temperature-dependent solid-state infrared spectroscopy ( Supplementary Figs 11 and 12 ) had shown that M0–M2 and D0–D2 were processable below their degradation temperature of 250 °C, and M2 and D2 exhibited detectable reversible thermal transitions associated to β-sheet deaggregation (at 170 °C and 178 °C according to DSC). In the following, we therefore decided to focus on blends of thermally processable materials, such as M2 , D1 and D2 , as well as unmodified polymers. All bulk materials were thoroughly thermally annealed at 120 °C for three days, which also served to remove residual traces of solvents. 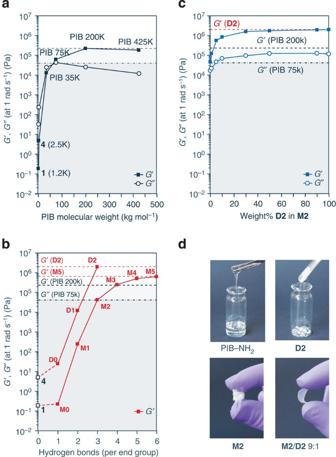Figure 4: Shear rheology on reinforced elastomers. Comparison of storage (G’) and loss moduli (G’’) at 1 rad s−1(a) of unmodified PIB as a function of molecular weight, (b) ofM0–M5andD0–D2as a function of hydrogen-bonding sites per end group and(c) of different blends ofM2/D2as a function of composition; the blends exhibited superior shear moduli compared with those of high molecular weight PIB even for low fractions ofD2. (d) Whereas the parent PIB amine was a viscous liquid,M2was a sticky solid,D2a brittle powder and a blend of 10 wt% ofD2inM2was an ‘inherently reinforced’ thermoplastic elastomer (Fig. 1c). SeeSupplementary Figs 7–10for more details on rheology measurements and temperature-dependent infrared spectroscopy. Figure 4: Shear rheology on reinforced elastomers. Comparison of storage ( G ’) and loss moduli ( G ’’) at 1 rad s −1 ( a ) of unmodified PIB as a function of molecular weight, ( b ) of M0–M5 and D0–D2 as a function of hydrogen-bonding sites per end group and (c ) of different blends of M2 / D2 as a function of composition; the blends exhibited superior shear moduli compared with those of high molecular weight PIB even for low fractions of D2 . ( d ) Whereas the parent PIB amine was a viscous liquid, M2 was a sticky solid, D2 a brittle powder and a blend of 10 wt% of D2 in M2 was an ‘inherently reinforced’ thermoplastic elastomer ( Fig. 1c ). See Supplementary Figs 7–10 for more details on rheology measurements and temperature-dependent infrared spectroscopy. Full size image Reinforced thermoplastic elastomers Independent of their composition, blends of M2 and D2 exhibited solid-state infrared spectra with amide I regions indistinguishable from the pure compounds ( Supplementary Fig. 13 ). The blends yielded materials with tailorable shear moduli that reached G′ =0.6 MPa on the addition of only about 5 wt% D2 and leveled off toward G′ ≈2 MPa for ≥10 wt% D2 , exceeding those of high MW PIB even for low fractions of D2 ( Fig. 4c,d and Supplementary Figs 9 and 10 ). At the same time, the materials underwent a sharp, single-step ‘melting’ transition at 160–170 °C associated with the deaggregation of all β-sheet structures according to temperature-dependent infrared spectroscopy ( Fig. 5a,b ), resulting in a drastic decrease of their moduli and viscosities ( Fig. 5c,d and Supplementary Fig. 14 ). The blends of mono- and difunctional derivatives with oligopeptide segments matching in length apparently became part of one and the same hydrogen-bonded network, resulting in PIB-based thermoplastic elastomers that were ‘inherently reinforced’ by the oligopeptide nanostructures ( Fig. 1c ). As a consequence, the blends M2 / D2 exhibited shear moduli one order of magnitude higher than those of even high MW PIB and, qualitatively, showed lower creep behaviour at room temperature. Moreover, both physical cross-links and reinforcing nanostructures melted simultaneously, yielding a sharp melting transition and well-processable melts with low viscosity at temperatures well below the materials’ decomposition. 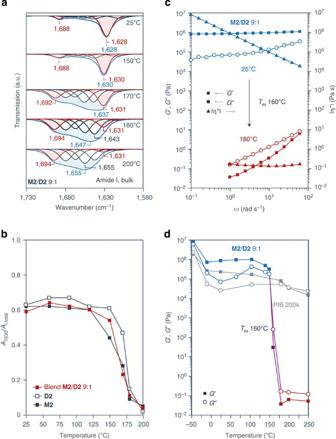Figure 5: Thermomechanical properties of reinforced elastomers. (a,b) Temperature-dependent infrared spectroscopy of the blendsM2/D29:1 wt% revealed a single-step ‘melting’ transition at 160–170 °C on heating, associated with the deaggregation of all β-sheet structures. (c) Shear rheology at different temperatures as well as (d) a plot ofG’andG’’at 1 rad s−1as a function of temperature (in comparison with high-molecular weight PIB) showed that the blendsM2/D29:1 wt% experienced a sharp decrease of their moduli at that temperature, yielding well-processable liquids. SeeSupplementary Figs 9–14for more details on rheology measurements and temperature-dependent infrared spectroscopy. Figure 5: Thermomechanical properties of reinforced elastomers. ( a , b ) Temperature-dependent infrared spectroscopy of the blends M2 / D2 9:1 wt% revealed a single-step ‘melting’ transition at 160–170 °C on heating, associated with the deaggregation of all β-sheet structures. ( c ) Shear rheology at different temperatures as well as ( d ) a plot of G’ and G’’ at 1 rad s −1 as a function of temperature (in comparison with high-molecular weight PIB) showed that the blends M2 / D2 9:1 wt% experienced a sharp decrease of their moduli at that temperature, yielding well-processable liquids. See Supplementary Figs 9–14 for more details on rheology measurements and temperature-dependent infrared spectroscopy. Full size image Interpenetrating supramolecular networks In contrast to the blends investigated above, we found polymer mixtures comprising ‘non-matching’ oligopeptides to give rise to separate hydrogen-bonded supramolecular aggregates and networks, producing novel ‘interpenetrating supramolecular networks’ with unusual thermomechanical properties ( Fig. 1d ). Thus, we investigated blends M2 / D1 in which the molecular structures of the two components were almost identical to the blends M2 / D2 but now featured two differently long oligopeptide segments. Binary blends of these materials were thermally annealed at 120 °C, which is below their melting transition at 139 °C but above the deaggregation temperature of D1 of 25–65 °C ( Supplementary Fig. 15 ). Whereas the pure β-sheet tape-forming M2 exhibited a gelation point in a classic rheological frequency sweep at 25 °C, the weakly aggregated but network-forming D1 exhibited properties very similar to PIB (MW 75,000 g mol −1 ), showing an entanglement point in the same frequency range at room temperature ( Supplementary Fig. 16 ). These rheological properties of the two components were superimposed in their blends, resulting in interesting materials with both a gelation and an entanglement point within a similar frequency range in a classical rheological frequency sweep at 25 °C. A blend of 20 wt% of M2 in D1 , for instance, exhibited a large frequency region with pronounced ‘liquid-like’ behaviour ( G″ > G′ ) at room temperature, confined by two regions of solid elastomer-like ( G′ > G″ ) behaviour at higher and lower shear frequencies, as seen from a rheological time-temperature superposition (TTS) master curve at 25 °C ( Fig. 6a ). High MW PIB materials may often exhibit such regions of ‘liquid-like’ behaviour at temperatures just above their glass transition temperature of T g ≈−60 °C ( Supplementary Fig. 17 ) [48] , [49] . However, the large temperature range at which this region was observed for the blend of M2 / D1 , its broad frequency range at room temperature and the extraordinarily large loss factor of up to tan δ =G″/ G′ =2.0 observed in this region are unprecedented in PIB-based materials. Hence, both the rheological and thermal properties of the blend M2 / D1 were completely different from those of the M2 / D2 (see above) despite their similar components, and although the former also contained partially stacked β-sheet tapes according to SAXS and WAXS ( Supplementary Fig. 18 ). On heating the blend M2 / D1 above the materials’ glass-transition temperature of T g =−55 °C, the storage and loss moduli first followed those of D1 ( Fig. 6b ); at about 65 °C, however, where pure D1 is already in its liquid regime according to DSC ( Supplementary Fig. 15 ), the storage and loss moduli became similar to those of M2 and remained constant up to the melting transition at above 139 °C. Although the apparent melting point depression as compared with pure M2 suggested some intermixing between D1 and M2 , the pronounced effect of the minority component M2 , the two-stage temperature transition (in contrast to the sharp, single-step melting of M2 / D2 at 160–170 °C) and the superimposed rheological properties of the individual components in the blend provide evidence for the presence of two independent hydrogen-bonded superstructures, resulting in an ‘interpenetrating supramolecular network’. 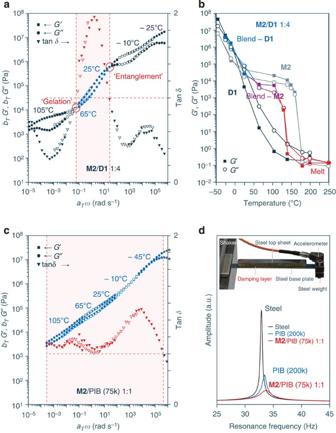Figure 6: Properties of interpenetrating supramolecular networks. (a) The rheological TTS master curve of a blendM2/D1(1:4) proved that the rheological features of its pure components were superimposed in the blend, resulting in a broad region with pronounced ‘liquid-like’ behaviour and a large loss factor of up to tanδ=2.0. (b) Temperature-dependent shear rheology of the blendM2/D1(1:4) in comparison with the pure components revealed that the material underwent a two-stage thermomechanical transition, following the behaviour ofD1in the temperature range of −55 °C to above room temperature, and thenM2between 65 °C and the melting transition at 139 °C. (c) According to the rheological TTS master curve ofM2/PIB (MW 75,000 g mol−1) (1:1), the materials had a loss factor of tanδ>0.6 over a very large frequency range. (d) Experimental setup for a random vibration modal analysis test on a sandwich structure comprising a damping layer. The first resonance frequency of the steel structure at 33 Hz and its intensity decrease in the sandwich structure for damping layers based on the blendM2/PIB (MW 75,000 g mol−1) (1:1) and unmodified PIB (MW 200,000 g mol−1). SeeSupplementary Figs 15–17andSupplementary Table 2for more details on shear rheology as well as shift factorsaTandbT. Figure 6: Properties of interpenetrating supramolecular networks. ( a ) The rheological TTS master curve of a blend M2 / D1 (1:4) proved that the rheological features of its pure components were superimposed in the blend, resulting in a broad region with pronounced ‘liquid-like’ behaviour and a large loss factor of up to tan δ =2.0. ( b ) Temperature-dependent shear rheology of the blend M2 / D1 (1:4) in comparison with the pure components revealed that the material underwent a two-stage thermomechanical transition, following the behaviour of D1 in the temperature range of −55 °C to above room temperature, and then M2 between 65 °C and the melting transition at 139 °C. ( c ) According to the rheological TTS master curve of M2 /PIB (MW 75,000 g mol −1 ) (1:1), the materials had a loss factor of tan δ >0.6 over a very large frequency range. ( d ) Experimental setup for a random vibration modal analysis test on a sandwich structure comprising a damping layer. The first resonance frequency of the steel structure at 33 Hz and its intensity decrease in the sandwich structure for damping layers based on the blend M2 /PIB (MW 75,000 g mol −1 ) (1:1) and unmodified PIB (MW 200,000 g mol −1 ). See Supplementary Figs 15–17 and Supplementary Table 2 for more details on shear rheology as well as shift factors a T and b T . Full size image Whereas the high-frequency boundary of the ‘liquid-like’ region can be assigned to the hydrogen-bonded supramolecular polymer formed by D1 and its entanglement, the low-frequency boundary can most probably be attributed to the secondary network formed by the M2 β-sheet tapes ( Fig. 1d ) that are entangled and partially aggregated into stacked superstructures, according to our SAXS and XRD results. Damping experiments As interpenetrating polymer networks bear significant potential in mechanical vibration damping applications [50] , [51] , the novel ‘interpenetrating supramolecular networks’ described here may provide an alternative avenue for the tailored preparation of high-performance damping materials. To this end, we investigated blends of M2 as an additive to unmodified PIB (MW 75,000 g mol −1 ). The latter had a molecular weight above its entanglement length and was chosen just because it had shown similar rheological properties as D1 (see above) under the same experimental conditions ( Supplementary Fig. 16 ). A mixture containing 50 wt% of M2 was shown to still contain the same partially stacked β-sheet tapes as pure M2 according to SAXS and WAXS ( Supplementary Fig. 18 ). The blend gave rise to a soft rubber-like material with storage and loss moduli G′ and G″ that were very similar to one another over almost the complete range of investigated frequencies, as determined from a TTS master curve at room temperature ( Fig. 6c ). As a result, the loss factor peaked at tan δ =1.1 at a reduced frequency a T ω =5 × 10 5 rad s −1 and never fell below tan δ =0.6 in the reduced frequency range of a T ω =10 −3 –10 6 rad s −1 . Moreover, the obtained master curves had a substantially different shape as compared with either pure M2 or unmodified PIB ( Supplementary Fig. 17 ); specifically, the rubbery plateau in the low-frequency regime was noticeably absent. By analogy to the example of the blend of D1 and M2 , we attributed these rheological features to an interpenetration of the network formed by the partially stacked M2 β-sheet tapes dispersed in the entanglement network of PIB (MW 75,000 g mol −1 ) that is similar to the one formed by D1 . If one uses the observed loss factor tan δ as a first-order indicator for damping properties, as it is often done in the pertinent literature [51] , [52] , the M2 /PIB blend ought to exhibit excellent damping performance over a broad frequency range. However, modal damping performance is actually the property of a system (that is, a base structure with damping treatment) and, as such, a complex function of different rheological parameters of all of its constituents and their geometry [53] . To quantitatively compare the performance of the M2 /PIB blend with other damping materials, we tested the shear vibration damping characteristics of the blend M2 /PIB (MW 75,000 g mol −1 ) (1:1) in comparison with high MW PIB (MW 200,000 g mol −1 ) [54] , [55] . We employed a random vibration modal analysis test on a sandwich structure representing a typical constrained damping layer application designed to investigate the structural damping performance in low-frequency vibration (30–40 Hz), as it is typical for the first vibration modes of steel or aluminum panels used in automotive or aerospace applications [42] . From the extent of the intensity decrease of the first resonance peak of the sandwich structure ( Fig. 6d ) compared with that of the steel structure alone, we calculated the modal damping ratios (obtained by a complex polynomial fraction fitting of the first peak of the frequency response function) to be ξ =2.7% for the blend M2 /PIB (MW 75,000 g mol −1 ) (1:1), which significantly exceeded the damping ratio of ξ =1.1% for unmodified PIB that is considered to possess good damping properties and is already used in damping applications on a technological scale [54] , [55] . Taking protein-based biomaterials as a model, the mono- and difunctional oligopeptide-modified PIBs and their blends investigated here constitute a versatile toolbox to obtain novel supramolecular materials with a broad range of mechanical properties. The oligopeptide end groups serve as multivalent hydrogen-bonded ligands but, in addition, show a distinct hierarchical structure formation. Our results prove that altering the length of the oligopeptide segments did not only result in the expected change in aggregation strength but also affected superstructure formation and nanoscopic morphology in a systematic way. Although our findings represent the first time that this feature has been systematically employed to tailor the bulk properties of polymers by oligopeptide modification, they can be straightforwardly rationalized using the well-understood models developed for the hierarchical self-organization of amyloidogenic oligopeptides [14] , [23] . According to these models, the molecular conformation in a β-strand conformation is twisted, resulting in β-sheet tapes with supramolecular helicity on hydrogen-bond-driven aggregation of the oligopeptides. It is this helical twisting of the constituting β-sheet tapes that self-limits lateral aggregation by β-sheet stacking into nanofibrils. As hydrogen-bonding in the hydrophobic PIB matrix is significantly stronger than in aqueous media, aggregation already occurs for relatively short oligo( L -alanine)s with n =2–5 alanine residues in the present case, and the relative differences in aggregation behaviour between the differently long oligopeptides are more drastic. Under these constraints, we reliably observed the formation of rigid, stacked β-sheet nanofibrils from M4 and M5 that had already been formed in solution and could not be thermally deaggregated in the bulk (below the decomposition temperature of the material). By contrast, M2–M3 did not aggregate in dilute solution but gave rise to extended β-sheet-like structures (single β-sheet tapes and stacked tape nanofibrils) with a sharp melting transition in bulk, supposedly formed under thermodynamic control in the course of solvent evaporation, when residual solvent still acted as a plasticizer. Finally, weak and undefined aggregates were thermally reversibly formed in the case of the short hydrogen-bonded end groups in bulk samples of M0–M1 . Moreover, we demonstrated for the first time that this selective, length-dependent self-assembly resulted in the formation of distinct nanostructures that coexisted even in bulk mixtures on annealing at a temperature chosen to be between the melting points of the pure components. Both the different solution-phase self-assembly properties and thermal transitions in bulk thus provided us with a handle to design supramolecular materials with vastly different mechanical properties from the same, limited number of constituent materials. More specifically, these features allowed us to simultaneously tailor the materials’ elastic properties and energy dissipation versus frequency. Thus, mixtures of mono- and difunctional compounds with oligopeptides matching in length, such as the mono- and difunctional dipeptide-substituted derivatives M2 and D2 , gave rise to supramolecular networks with tunable cross-linking density. These networks were, at the same time, inherently reinforced by the extended β-sheet aggregates (tapes and nanofibrils). These aggregates may themselves be regarded as sufficiently stable supramolecular polymers to give rise to an entanglement network. In these materials, the difunctional compound D2 supposedly serves as an additional cross-linker that prevents slipping of the tapes and nanofibrils. As a result, we obtained elastomers with low loss factor, low creep and moduli that were already superior to those of the unmodified high MW polymers, even at a low content of the difunctional cross-linker. As both physical cross-links and reinforcing nanostructures were part of one and the same hydrogen-bonded network, both melted at the same sharp transition temperature, resulting in well-processable melts of low viscosity. By contrast, blends of mono- and difunctional compounds with oligopeptides not matching in length were found to form novel ‘interpenetrating supramolecular networks’ from segregated β-sheet aggregates and hydrogen-bonded networks. As a result, even materials that were chosen to be as similar as possible in molecular structure and composition to the blends with matching oligopeptides (such as blends M2 / D1 , compared with the previous blends M2 / D2 ) had significantly different thermomechanical properties. In particular, the energy dissipation properties of the blends, as well as their frequency and temperature dependence, could be tailored in a broad manner, even if the individual components had very similar rheological properties (such as for the blends M2 /PIB (MW 75,000 g mol −1 ) compared with the previous blends M2 / D1 ). As a result, some of the obtained materials displayed a very large loss factor at a temperature well below their melting transition and different from the constituent polymer’s glass transition. These features may be of interest in terms of self-healing applications, as the materials bear a resemblance to previously investigated self-healing elastomers [41] , in that they combine dynamic network formation with high diffusivity below their melting temperature. On the other hand, blends of our materials with unmodified polymers exhibited a large loss factor over the whole investigated frequency range and were indeed found to exhibit excellent properties in constrained layer damping that are relevant to several fields of current technology, such as automotive and aerospace engineering [42] . The different shape of the TTS master curves of the blends compared with their pure components indicated that neither do the tapes formed by M2 just serve as a filler nor does the PIB matrix just act as a diluting ‘solvent’. Rather, the resulting supramolecular network of the tapes with large fractions of ‘pendant’ polymer chains well dispersed in the matrix (of the same polymer material) is conceptually related to damping materials based on ‘irregular’ poly(siloxane) networks, in which the damping performance was attributed to improved energy dissipation by the high fraction of such ‘pendant’ polymer chains incorporated into the network [56] . It is worth noting that the obtained damping performance of the investigated blends already matches that of typical commercial high-performance damping materials that are usually complex formulations of a polymer matrix, additives and fillers. This renders such blends attractive matrix materials in nanocomposites for use in high-performance damping materials. In conclusion, the self-sorting aggregation of short oligopeptide end groups placed in a hydrophobic polymer matrix into different types of nanostructures and superstructures has provided us with a toolbox to obtain materials with a broad variety of properties, ranging from reinforced elastomers to soft damping materials. We think that this versatility will be relevant to the design of novel elastomer materials with unusual thermomechanical property profiles, such as frequency-dependent but temperature-invariant energy dissipation. General A comprehensive account of all methods, including instrumentation, materials, syntheses and analytical data of M0–M5 and D0–D5 , as well as their mass and NMR spectra ( Supplementary Figs 19–36 ) can be found in the Supplementary Information . Atomic force microscopy AFM imaging was performed on a Nanoscope IIIa instrument. Samples were prepared from stock solutions of the compounds in tetrachlorethane at an initial concentration c= 10 −3 mol l −1 . The solutions were placed into sealed tubes, vigorously stirred (400 r.p.m.) and heated in an oil bath to 180 °C for 2 h, followed by stepwise cooling 160 °C (1 h), 140 °C (1 h), 120 °C (1 h) and 100 °C (1 h) under continued stirring (100 r.p.m.). Afterwards, the heating was switched off and the solution was allowed to cool to room temperature at the same stirring rate. The solutions were then diluted to a concentration of c= 1·10 −4 mol l −1 or c= 5·10 −5 mol l −1 and spin-coated onto SiO 2 substrates treated with ethanol and ultrapure water (3,000 r.p.m.) or onto freshly cleaved HOPG (1,800 r.p.m.). The obtained samples were analysed in tapping mode at room temperature in air, using cantilevers with an average resonance frequency of 75 kHz and scan rates of 0.5–1.5 Hz. The image resolution was 512 × 512 pixels. X-ray diffraction XRD measurements were performed on a PANalytical X’Pert Pro diffractometer in conventional Bragg-Brentano θ −2 θ geometry with a 240-mm goniometer radius. CuKα X-rays were generated using 40 mA and 45 kV operating conditions. Incident beam Soller slits of 0.04 rad were used, and the incident divergence and antiscatter slits were fixed at 0.5°. Air scattering was reduced using a beam knife. The receiving antiscatter slit was fixed at 1° and receiving Soller slits limiting the axial divergence to 0.04 rad were positioned in the diffracted beam path. An X’Celerator linear position-sensitive X-ray detector with a length of 2.122 °2 θ was used for data acquisition. All scans were measured over an angular range of 2 θ =5–30° with 0.017° step size and accumulated time per step of 180 s, resulting in a total measurement time of about 38 min per scan. Small-angle X-ray scattering SAXS was performed with a Rigaku S-MAX3000 pinhole camera (Rigaku Innovative Technologies, Auburn Hills, USA). The samples were kept in vacuum at room temperature during the measurements. The scattering data were presented as a function of the scattering vector modulus q =4 π / λ sin( θ /2), where θ is the scattering angle and λ is the photon wavelength. The same monochromatized CuKα radiation was used as in the XRD instrument. Dynamic shear rheology Dynamic shear rheology experiments were carried out on parallel plate rheometers AR 2000, ARES LR2 or ARES from TA Instruments. Disc-shaped sample specimen from all materials that were shape-persistent were prepared on a Rittal table press. A force of 2 kN was applied for 30 min at 100 °C, after which the specimen were cooled to 20 °C at a force of 1.1 kN for 30 min. Depending on the samples quantity, aluminum plates of 15- or 25-mm diameter, as well as stainless steel plates of 25-mm diameter were used. Discs of 12-mm diameter were prepared as well and placed in the centre of the stainless steel plates (25-mm diameter) with a centring tool. The gap between the plates was in the range of 0.4–2 mm. In the case of non-adhesive samples, the plates were covered with emery paper to avoid wall slipping. Measurements were carried out at temperatures of −45 °C to 250 °C. Once the desired temperature was reached, the system was equilibrated for 2 min. Frequency sweeps ranging from 100 to 0.01 rad s −1 were carried out under controlled strain. Depending on the sample composition and temperature, the strain amplitude ranged from 0.03% to 50%. The applied strain was defined such that the sample stayed in its linear viscoelastic domain during the complete frequency sweep. Modal damping tests Constrained layer damping tests were carried out on a RMS 3000 vibration shaker using an HP 35670A vibration controller and signal analyser in open-loop pseudo-random vibration analysis. The acceleration of the base and of the tip of the specimen were monitored using two Bruel&Kaer 4,517 accelerometer through a B&K Nexus 2,692 amplifier. The frequency transfer functions of the different specimens were measured in a frequency range of 10–110 Hz with a resolution of 0.125 Hz. The test specimen consisted of a sandwich structure representing a constrained damping layer application. The base substrate was a steel plate with dimensions of 60 × 6 × 0.5 mm onto which a damping layer with dimensions of 40 × 6 × 2.0 mm was superimposed. A thin steel plate with dimensions of 40 × 6 × 0.2 mm was used to constrain the top of the damping layer. The sandwich test structure was then clamped with one end to the vibration table over a length of 6 mm, and a mass of 4.6 g was added to the free end of the beam over a length of 5 mm. The added mass has been calculated such that the first bending mode of the sandwich beam is in the range of 30–40 Hz. To determine the modal damping ratio ξ , the first peak of the frequency response function was first fitted using a complex polynomial fraction least-square method integrated in the HP 35670A signal analyser. The modal damping ratio ξ was then calculated from the real part λ and the imaginary part ω of the first complex pole of the polynomial fraction using the definition ξ = λ / ω . Sample preparation For the preparation of films and solid samples of either single compounds or blends, the oligopeptide-polymer derivatives and/or PIB (MW 75,000 g mol −1 ) were dissolved in either tetrachlorethane or CHCl 3 , the solutions were stirred at room temperature for 1–16 h and concentrated in vacuo . The resulting materials were dried in high vacuum at 120 °C for 3 days. How to cite this article: Croisier, E. et al. A toolbox of oligopeptide-modified polymers for tailored elastomers. Nat. Commun. 5:4728 doi: 10.1038/ncomms5728 (2014).